O-GlcNAc-mediated interaction between VER2 and TaGRP2 elicitsTaVRN1mRNA accumulation during vernalization in winter wheat Vernalization, sensing of prolonged cold, is important for seasonal flowering in eudicots and monocots. While vernalization silences a repressor (FLC, MADS-box transcription factor) in eudicots, it induces an activator (TaVRN1, an AP1 clade MADS-box transcription factor) in monocots. The mechanism for TaVRN1 induction during vernalization is not well understood. Here we reveal a novel mechanism for controlling TaVRN1 mRNA accumulation in response to prolonged cold sensing in wheat. The carbohydrate-binding protein VER2, a jacalin lectin, promotes TaVRN1 upregulation by physically interacting with the RNA-binding protein TaGRP2. TaGRP2 binds to TaVRN1 pre-mRNA and inhibits TaVRN1 mRNA accumulation. The physical interaction between VER2 and TaGRP2 is controlled by TaGRP2 O -GlcNAc modification, which gradually increases during vernalization. The interaction between VER2 and O -GlcNAc-TaGRP2 reduces TaGRP2 protein accumulation in the nucleus and/or promotes TaGRP2 dissociation from TaVRN1 , leading to TaVRN1 mRNA accumulation. Our data reveal a new mechanism for sensing prolonged cold in temperate cereals. Many plants that grow in temperate climates, including the temperate cereals (such as wheat and barley) and dicot species (such as Arabidopsis ), need exposure to prolonged cold during the winter to flower in the spring, a process termed vernalization [1] . This helps to ensure reproductive success by reducing the likelihood of cold-sensitive floral organs being damaged by winter frost or of reduced fertility due to heat and water stress during summer [2] , [3] . Various categories of genes controlling vernalization-induced flowering have been identified in the model plant Arabidopsis and the cereal crops wheat and barley [4] , [5] , [6] , [7] , [8] , [9] , [10] . In Arabidopsis , vernalization results in transcriptional and Polycomb-mediated downregulation of a potent flowering repressor, the MADS-box transcription factor flowering locus C (FLC) [4] , [9] , [11] . However, cereals do not contain a homologue of FL C, and genetically defined vernalization-related genes ( TaVRN1-3 ) in wheat are quite different from their counterparts in Arabidopsis , suggesting that the vernalization response may have evolved independently in dicotyledonous and monocotyledonous plants [10] , [11] . TaVRN1 acts as a major flowering promoter that mediates vernalization-induced flowering in cereals [5] , [6] , [7] . It encodes a MADS-box transcription factor with high similarity to the Arabidopsis meristem-identity genes AP1 , CAL and FRUITFULL [5] , [6] , [7] . TaVRN1 transcripts are present at very low basal levels before vernalization but increase gradually during prolonged cold exposure in the shoot apex and leaf in a quantitative manner, with longer cold treatment inducing higher transcript level [5] , [6] , [7] , [8] . TaVRN1 may have distinct roles in the shoot apex and the leaf. In the shoot apex, TaVRN1 is likely to affect the transition from the vegetative phase to infloresence, whereas in the leaf it is thought to facilitate long-day induction of TaVRN3 ( Arabidopsis FT homologue) by downregulating the expression of the flower repressor TaVRN2 (a ZCCT domain-containing protein) [10] , [12] . Elevated expression of TaVRN1 is maintained in the shoot apex and leaves after vernalization, and the accumulation of TaVRN1 mRNA in these organs may determine how rapidly plants flower [8] , [10] , [12] . However, how TaVRN1 expression is activated during vernalization remains not well understood. Vernalization, as a seasonal environmental stimulus, shapes the metabolic patterns of carbohydrate and nitrogen in wheat and cauliflower, thus changing the cellular nutrient status [13] , [14] . O -GlcNAcylation is a post-translational modification sensitive to the cellular nutrient status [15] . Two conserved enzymes, O -GlcNAc transferase (OGT) and O -GlcNAcase (OGA), mediate the reversible addition and removal of a single O -linked-β-N-acetylglucosamine ( O -GlcNAc) to the hydroxyl groups of serine and/or threonine residues of substrate proteins [16] , [17] . Over 1,000 proteins are known to be O -GlcNAcylated, with O -GlcNAc modification of cytosolic and nuclear proteins affecting their localization, phosphorylation, interaction with other proteins and/or stability [17] . In animals, O -GlcNAc controls diverse aspects of cell physiology in different tissue types, and O -GlcNAc signalling is implicated in human diseases such as type II diabetes and neurodegeneration [18] , [19] , [20] . In plants, the A. thaliana genome encodes two putative OGTs, SPINDLY (SPY) and SECRET AGENT (SEC). They have overlapping functions in gametes and during embryogenesis [21] , [22] . In addition, sec mutants show subtle growth defects, whereas SPY is known to function in the gibberellin, cytokinin, red light response and circadian pathways [23] , [24] . SPY interacts with and may modify a TCP family transcription factor to promote cytokinin responses in leaves and flowers [25] . Other types of plant proteins that are O -GlcNAcylated include nuclear pore complex components and histone proteins [26] , [27] . Currently, a major challenge in plant biology is to elucidate how O -GlcNAc signalling responds to environmental stimuli and affects plant development. Previously, we cloned a vernalization-induced gene called vernalization-related 2 ( VER2 ) by mRNA differential display from hexaploid winter wheat [28] . The VER2 transcript level significantly influences flowering as well as spikelet development [29] . VER2 encodes a nucleocytoplasmic carbohydrate-binding protein, a jacalin-like lectin, with high affinity for GlcNAc and galactose [30] . In response to vernalization, VER2 accumulates predominantly in the nucleus in shoot tips and young leaves, but also weakly in the cytoplasm [30] . O -GlcNAc-modified proteins are specifically recognized by VER2 in vernalized wheat plants, and global O -GlcNAcylation levels increase during vernalization and decrease after de-vernalization (a subsequent high-temperature treatment following the cold treatment) [30] . However, the O -GlcNAc-modified targets of VER2 that mediates flowering in response to prolonged cold are still unknown. Here we report that the RNA-binding protein TaGRP2 is O -GlcNAc modified in response to vernalization. TaGRP2 inhibits transcript accumulation of the key flowering-promoting gene, TaVRN1 , by directly binding to a winter variety ‘critical region’ located in the first intron of the TaVRN1 pre-mRNA. During vernalization, nuclear-localized VER2 interacts with O -GlcNAc-modified TaGRP2 to relieve the repression on TaVRN1 transcript accumulation and to promote flowering in hexaploid winter wheat. Jacalin lectin VER2 accelerates flowering in hexaploid wheat Previously, we cloned the vernalization-induced gene VER2 (ref. 28 ), here we use fluorescence in situ hybridization assays to identify its chromosome localization. On the basis of the multicolour-labelled (pAs1 for red and pSc119.2 for green) chromosome profile, signal for VER2 probe, labelled with Alexa Fluor-488-5-dUTP, was only detected on the long arm of chromosome 2D ( Supplementary Fig. 1a ). Consistent with this, genome sequence alignment showed that VER2 is a unique gene located on the scaffold 10222 of Chromosome 2D ( Supplementary Fig. 1b ) [31] . We had previously reported that knockdown of VER2 by antisense RNA causes delayed flowering and reduced heading [29] . By contrast, VER2 -overexpression ( VER2 -OE) lines in the JH9 accession (a local hexaploid winter wheat cultivar with a strong requirement for vernalization) were earlier flowering and had elevated heading compared with wild type in the field ( Fig. 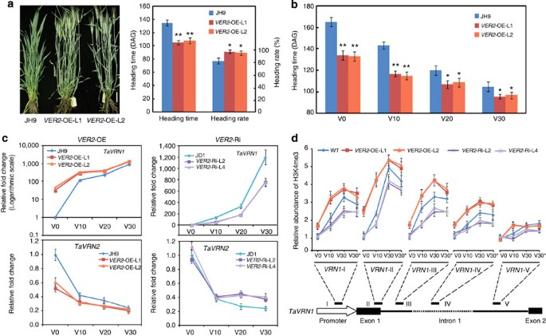Figure 1: VER2 influencesTaVRN1expression and accelerates flowering. (a) Morphological phenotype (110 DAG) and heading time or heading rate (130 DAG) ofVER2-OE transgenic wheat compared with wild-type JH9 under natural vernalization in the field (in Bashang, Hebei province, China). DAG, day after germination; data are means±s.d. of 30 plants for each line. Student’st-test showed the statistical significance, *P<0.05; **P<0.01. Scale bar, 5 cm. (b) Heading time ofVER2-OE transgenic wheat compared with wild-type JH9 in the greenhouse under long-day (16 h light/8 h dark) condition after different days of cold exposure, data shown are mean±s.d. of 30 plants for each line. Student’st-test showed the statistical significance, *P<0.05; **P<0.01. (c) Transcript level of the key flowering genesTaVRN1andTaVRN2inVER2-OE,VER2-Ri and wild-type JH9 or JD1 plants (normalized toTubulin). The expression levels ofTaVRN1andTaVRN2in wild-type JH9 or JD1 at V0 (non-vernalized plant, grown in long-day condition at 20 °C for 5 days) are set as 1. Relative expression fold change in transgenic plants after different cold exposure is shown. V10–30, plants are grown in long-day conditions at 22 °C for 3 days, then transferred to 4 °C for 10–30 days, above ground part of 15 seedlings per sample were collected at 4 °C for RNA extraction. Data are means±s.d. of three parallel samples. (d) Histone modification (H3K4me3) atTaVRN1chromatin loci during the course of vernalization inVER2-OE,VER2-Ri and wild-type JH9 or JD1. The regions amplified (I–V) after ChIP is shown in the schematic diagram of theTaVRN1gene structure. The data were first normalized to input sample, then normalized toACTIN. The amounts of precipitated DNA in wild-type (WT) JH9/JD1 at V0 were set as 1 and relative fold changes in transgenic plants compared with wild type under different cold exposure times are given. Data are means±s.d. of three parallel samples. V30* means V30 vernalization treatment followed by normal temperature (20 °C) growth for 2 days. 1a ; Supplementary Table 1 ). The accelerated-flowering phenotype of VER2 -OE relative to JH9 was gradually reduced by prolonged cold treatment ( Fig. 1b ; Supplementary Table 1 ), suggesting that VER2 mainly functions in the vernalization pathway to promote flowering. Figure 1: VER2 influences TaVRN1 expression and accelerates flowering. ( a ) Morphological phenotype (110 DAG) and heading time or heading rate (130 DAG) of VER2 -OE transgenic wheat compared with wild-type JH9 under natural vernalization in the field (in Bashang, Hebei province, China). DAG, day after germination; data are means±s.d. of 30 plants for each line. Student’s t -test showed the statistical significance, * P <0.05; ** P <0.01. Scale bar, 5 cm. ( b ) Heading time of VER2 -OE transgenic wheat compared with wild-type JH9 in the greenhouse under long-day (16 h light/8 h dark) condition after different days of cold exposure, data shown are mean±s.d. of 30 plants for each line. Student’s t -test showed the statistical significance, * P <0.05; ** P <0.01. ( c ) Transcript level of the key flowering genes TaVRN1 and TaVRN2 in VER2 -OE, VER2 -Ri and wild-type JH9 or JD1 plants (normalized to Tubulin ). The expression levels of TaVRN1 and TaVRN2 in wild-type JH9 or JD1 at V0 (non-vernalized plant, grown in long-day condition at 20 °C for 5 days) are set as 1. Relative expression fold change in transgenic plants after different cold exposure is shown. V10–30, plants are grown in long-day conditions at 22 °C for 3 days, then transferred to 4 °C for 10–30 days, above ground part of 15 seedlings per sample were collected at 4 °C for RNA extraction. Data are means±s.d. of three parallel samples. ( d ) Histone modification (H3K4me3) at TaVRN1 chromatin loci during the course of vernalization in VER2 -OE, VER2 -Ri and wild-type JH9 or JD1. The regions amplified (I–V) after ChIP is shown in the schematic diagram of the TaVRN1 gene structure. The data were first normalized to input sample, then normalized to ACTIN . The amounts of precipitated DNA in wild-type (WT) JH9/JD1 at V0 were set as 1 and relative fold changes in transgenic plants compared with wild type under different cold exposure times are given. Data are means±s.d. of three parallel samples. V30* means V30 vernalization treatment followed by normal temperature (20 °C) growth for 2 days. Full size image We next compared the expression of the vernalization gene TaVRN1 in JH9 and VER2 -OE plants. Transcript abundance of TaVRN1 was increased in VER2 -OE lines compared with the wild-type JH9 at the seedling stage ( Fig. 1c ). Of note, without cold exposure (V0), the increase in TaVRN1 transcript level in VER2 -OE lines relative to JH9 was more dramatic, consistent with the more significant acceleration of the flowering transition phenotype ( Fig. 1b ). Expression of the TaVRN2 gene, a repressor of flowering, showed the opposite pattern to TaVRN1 in the VER2 -OE transgenic lines ( Fig. 1c ), consistent with the previously suggested negative regulation of TaVRN2 transcription by TaVRN1 (refs 32 , 33 ). In VER2 RNAi interference ( VER2 -Ri) lines, TaVRN1 expression was downregulated compared with wild-type JD1, with remarkable decrease in expression after prolonged (V10, V20, V30) cold exposure (4 °C) while TaVRN2 expression was increased ( Fig. 1c ). During vernalization, the histone modification status dynamically changed at the TaVRN1 locus, consistent with the increased TaVRN1 transcription level [34] , [35] . In agreement with the observed increase in TaVRN1 mRNA accumulation, the activating histone H3 modification H3K4me3 increased at this locus in VER2 -OE lines, particularly at the promoter and in first intron before (V0), during (V10, V30) and after cold exposure (V30+2) compared with wild type, with opposite changes in VER2 -Ri lines ( Fig. 1d ). Thus, VER2 may act upstream of TaVRN1 to accelerate flowering in winter wheat during vernalization. TaGRP2 interacts with VER2 and regulates flowering in wheat Given that VER2 encodes a lectin, it may work in concert with other factors to influence TaVRN1 expression level. To screen for VER2 interactors, total proteins extracted from vernalized plumules were fractionated using ion-exchange chromatography followed by gel filtration chromatography. Fractions containing potential VER2-interacting proteins (VIPs) were tracked by immunoblotting with VER2 antibody. The proteins co-segregating with VER2 were separated by SDS–polyacrylamide gel electrophoresis (PAGE), and further characterized by mass spectrometry (MS; Fig. 2a ). 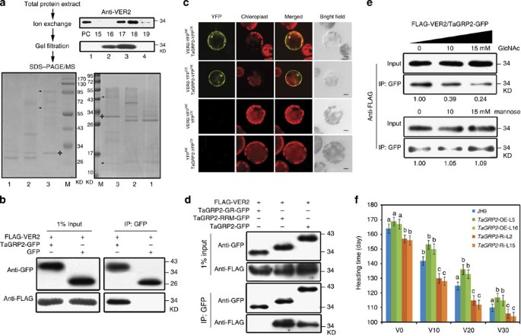Figure 2: TaGRP2 interacts with VER2 and regulates flowering time. (a) Chromatographic isolation and MS identification of VER2-co-segregating proteins after vernalization treatment. Different fractions from the ion-exchange and gel filtration chromatography were immunoblotted with anti-VER2 antibody. The SDS–PAGE shows the fractions (1–3) from the gel filtration. Black arrowhead indicates the protein band identified by MS. ‘+’ shows the VER2 protein band. PC, positive control for immunobloting. (b,c) Co-IP and BiFC assays to confirm the interaction between VER2 and TaGRP2. Scale bar, 10 μm. (d) Co-IP assay indicating that the RRM domain mediates the interaction between TaGRP2 and VER2. (e) GlcNAc pre-incubation reduced the interaction between VER2 and TaGRP2. The relative intensity (IP/input) was quantified using Image J. (f) Heading time ofTaGRP2-OE,TaGRP2-Ri and JH9 plants after different periods of cold exposure, data are means±s.d. of 30 plants for each line. Statistical analyses of multiple comparisons were done by Tukey’s honestly significant difference (HSD) test; different characters indicate statistically significant differences within groups. In total, we identified nine potential VIPs ( Supplementary Table 2 ). One of them, VIP2, is a member of the highly conserved glycine-rich RNA-binding protein (GRP or GR-RBP) family [36] , [37] , TaGRP2, and is an orthologue of Arabidopsis AtGRP7, which functions in regulation of FLC transcript level and flowering time ( Supplementary Fig. 2 ) [38] . An HvGR-RBP1-containing locus on barley ( Hordeum vulgare L.) chromosome 6 was reported to influence flowering time and leaf senescence [39] . Therefore, we chose TaGRP2 for further analysis. Figure 2: TaGRP2 interacts with VER2 and regulates flowering time. ( a ) Chromatographic isolation and MS identification of VER2-co-segregating proteins after vernalization treatment. Different fractions from the ion-exchange and gel filtration chromatography were immunoblotted with anti-VER2 antibody. The SDS–PAGE shows the fractions (1–3) from the gel filtration. Black arrowhead indicates the protein band identified by MS. ‘+’ shows the VER2 protein band. PC, positive control for immunobloting. ( b , c ) Co-IP and BiFC assays to confirm the interaction between VER2 and TaGRP2. Scale bar, 10 μm. ( d ) Co-IP assay indicating that the RRM domain mediates the interaction between TaGRP2 and VER2. ( e ) GlcNAc pre-incubation reduced the interaction between VER2 and TaGRP2. The relative intensity (IP/input) was quantified using Image J. ( f ) Heading time of TaGRP2 -OE, TaGRP2 -Ri and JH9 plants after different periods of cold exposure, data are means±s.d. of 30 plants for each line. Statistical analyses of multiple comparisons were done by Tukey’s honestly significant difference (HSD) test; different characters indicate statistically significant differences within groups. Full size image We used co-immunoprecipitation (Co-IP) and bimolecular fluorescence complementation (BiFC) assays to probe the interaction between VER2 and TaGRP2. FLAG-VER2 was co-expressed with TaGRP2-GFP or GFP alone in protoplasts of vernalized wheat plumules. After IP with a GFP antibody, FLAG-VER2 was detected in the immunoprecipitate of the FLAG-VER2/TaGRP2-GFP co-expression line, but not in that from the FLAG-VER2/GFP line, suggesting that VER2 and TaGRP2 interacted in plant cells ( Fig. 2b ). BiFC assays confirmed the physical interaction and revealed that it occurred both in the nucleus and in the cytoplasm ( Fig. 2c ). Domain-deletion assays showed that the RNA recognition motif (RRM)-containing domain of TaGRP2, but not its glycine-rich domain, was required for the interaction with VER2 ( Fig. 2d ). Notably, the interaction between VER2 and TaGRP2, as observed by Co-IP, was reduced about 60–75% in the presence of exogenous GlcNAc in a dose-dependent manner, whereas addition of mannose at the same concentrations caused nearly no change ( Fig. 2e ). The combined data suggest that the carbohydrate-binding ability of the lectin protein VER2 may be involved in its physical interaction with TaGRP2. To assess whether TaGRP2 is a biological relevant interactor of VER2 during vernalization, TaGRP2 overexpression and knockdown wheat plants were generated in the JH9 background by microprojectile bombardment-mediated transformation [40] . The TaGRP2 -OE lines showed delayed flowering, whereas TaGRP2 -Ri plants accelerated flowering compared with wild type. In addition, the delayed flowering time of TaGRP2 -OE was reduced by prolonged exposure to cold ( Fig. 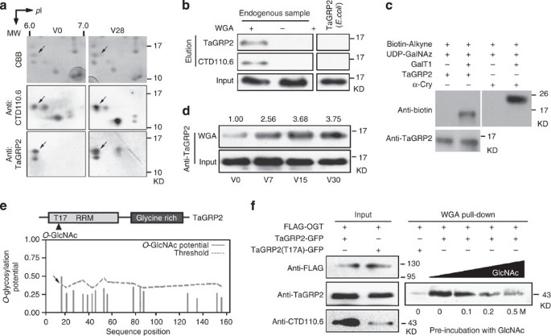Figure 3: Vernalization regulates dynamicO-GlcNAcylation status of TaGRP2. (a) Endogenous TaGRP2 isO-GlcNAcylated. 2D PAGE was used to separate total protein extracted from wheat plumules, followed by immunoblotting with antibodies against TaGRP2 or Thr/Ser-O-GlcNAcylated proteins (Anti-CTD110.6). Arrows indicate the TaGRP2 protein spot characterized by MS. V0, non-vernalized sample; V28, 28 days’ 4 °C vernalized sample; CBB, Coomassie Brilliant Blue staining. (b) WGA affinity purification of endogenousO-GlcNAcylated TaGRP2 protein, but notE. coli-expressed TaGRP2. (c) Detection ofO-GlcNAc-modified TaGRP2. Endogenous TaGRP2 was affinity purified by TaGRP2 antibody followed by labelling in the presence of UDP-GalNAz and reacted with TAMRA alkyne for detection by anti-biotin. α-Cry protein serves as positive control. (d) TaGRP2 isO-GlcNAcylated during vernalization (V0, non-vernalized; V7, V15 and V30, 7, 15 and 30 days’ 4 °C vernalized sample). WGA was used to affinity purifyO-GlcNAcylated proteins, and then immunoblot to detect TaGRP2 using anti-TaGRP2 antibody. Numbers above indicate relative intensity (WGA/input) as quantified using Image J. (e) Prediction of theO-GlcNAcylation site in TaGRP2 by YinOYang online prediction toolhttp://www.cbs.dtu.dk/services/YinOYang/. (f) Point mutation of Thr17 dramatically reduced the level ofO-GlcNAcylation of TaGRP2. 2f ; Supplementary Table 3 ). The data are consistent with the notion that TaGRP2 is a flowering repressor with a role in vernalization in winter wheat. In summary, VER2 interacts with the flowering repressor TaGRP2 during vernalization in winter wheat, and this interaction is mediated by the RRM domain of TaGRP2 and the carbohydrate-binding domain of VER2. TaGRP2 is dynamically O -GlcNAcylated during vernalization Previous findings that VER2 may interact with O -GlcNAcylated proteins after vernalization [30] , together with the current evidence that exogenous GlcNAc addition attenuated the interaction between VER2 and TaGRP2, suggested the possibility that TaGRP2 might be O -GlcNAc modified during vernalization. To address this possibility, total protein from wheat plumules was separated using two-dimensional gel electrophoresis and visualized by immunoblotting with CTD110.6 antibody, which could recognize Thr/Ser O -GlcNAcylation in proteins, as well as with a TaGRP2-specific antibody. The same spot was detected by the CTD110.6 antibody and by the TaGRP2 antibody ( Fig. 3a ), and MS confirmed that this spot corresponds to TaGRP2. In a complementary approach, we used wheat germ agglutinin (WGA, with ability to bind N-acetyl-D-glucosamine) for affinity purification of total lysates from plumules and probed the precipitate with TaGRP2 antibody and CTD110.6. We successfully detected O -GlcNAcylated endogenous TaGRP2 in the bound fraction after elution ( Fig. 3b ). As a negative control, recombinant TaGRP2 from Escherichia coli was used. No signal was detected by either TaGRP2 or CTD110.6 antibody after WGA purification ( Fig. 3b ). To exclude the possibility of non-specific recognition by WGA and/or CTD110.6 (ref. 41 ), a commercial highly specific detection system (Click-iT Protein Analysis Detection Kits, Invitrogen) [42] , based on the specific attachment of azido-modified galactose (GalNAz) to O -GlcNAc residues on target proteins, was used to determine whether endogenous TaGRP2 was O -GlcNAcylated. TaGRP2 protein was enriched and purified from wheat plumules after vernalization treatment by affinity chromatography, then labelled and detected ( Supplementary Fig. 3 ). TaGRP2 could be detected by anti-biotin antibody, as could the positive control protein α-crystallin, after specific labelling of the GlcNAc moiety ( Fig. 3c ). The combined data suggested that endogenous TaGRP2 is O -GlcNAc modified. Consistent with the previous finding that global O -GlcNAc modification levels increased with vernalization treatment [30] , the amount of O -GlcNAcylated TaGRP2 progressively increased over the course of vernalization ( Fig. 3d ). Figure 3: Vernalization regulates dynamic O -GlcNAcylation status of TaGRP2. ( a ) Endogenous TaGRP2 is O -GlcNAcylated. 2D PAGE was used to separate total protein extracted from wheat plumules, followed by immunoblotting with antibodies against TaGRP2 or Thr/Ser- O -GlcNAcylated proteins (Anti-CTD110.6). Arrows indicate the TaGRP2 protein spot characterized by MS. V0, non-vernalized sample; V28, 28 days’ 4 °C vernalized sample; CBB, Coomassie Brilliant Blue staining. ( b ) WGA affinity purification of endogenous O -GlcNAcylated TaGRP2 protein, but not E. coli -expressed TaGRP2. ( c ) Detection of O -GlcNAc-modified TaGRP2. Endogenous TaGRP2 was affinity purified by TaGRP2 antibody followed by labelling in the presence of UDP-GalNAz and reacted with TAMRA alkyne for detection by anti-biotin. α-Cry protein serves as positive control. ( d ) TaGRP2 is O -GlcNAcylated during vernalization (V0, non-vernalized; V7, V15 and V30, 7, 15 and 30 days’ 4 °C vernalized sample). WGA was used to affinity purify O -GlcNAcylated proteins, and then immunoblot to detect TaGRP2 using anti-TaGRP2 antibody. Numbers above indicate relative intensity (WGA/input) as quantified using Image J. ( e ) Prediction of the O -GlcNAcylation site in TaGRP2 by YinOYang online prediction tool http://www.cbs.dtu.dk/services/YinOYang/ . ( f ) Point mutation of Thr17 dramatically reduced the level of O -GlcNAcylation of TaGRP2. Full size image Scanning TaGRP2 for a possible O -GlcNAc target site, we identified Thr17 in the RRM domain of TaGRP2 as a potential O -GlcNAc site ( Fig. 3e ). To test the importance of this site, we mutagenized TaGRP2 Thr17 to Ala17 and co-expressed it with FLAG-tagged human OGT [43] in tobacco leaves. Immunoblotting with the CTD110.6 antibody showed that the mutant had markedly reduced O -GlcNAcylation ( Fig. 3f ). Similar patterns appeared in WGA affinity purification assays ( Fig. 3f ). However, O -GlcNAc modification was not abolished in TaGRP2m T17A , indicating that other O -GlcNAc modification sites may exist in TaGRP2. We conclude that vernalization regulates the O -GlcNAc modification status of TaGRP2, and that Thr17 is one of the sites of modification of TaGRP2. O -GlcNAcylation of TaGRP2 influences its characteristics We next asked whether the O -GlcNAc modification of TaGRP2 is of functional significance. PUGNAc, an inhibitor of OGA [44] , was used to elevate the cellular O -GlcNAc modification levels ( Supplementary Fig. 4 ). PUGNAc treatment increased the amount of FLAG-VER2 co-immunoprecipitated with TaGRP2-GFP ( Fig. 4A ). By contrast, the point mutant TaGRP2m T17A reduced interaction with VER2 relative to wild-type TaGRP2. In addition, neither GlcNAc pre-incubation nor PUGNAc treatment changed the interaction intensity between VER2 and TaGRP2m T17A ( Fig. 4B ). This suggests that O -GlcNAc modification at Thr17 of TaGRP2 may be important for its interaction with VER2. 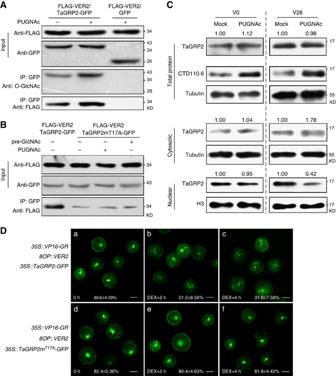Figure 4:O-GlcNAcylation of TaGRP2 influences its characteristics. (A,B) VER2 predominantly interacts withO-GlcNAcylated TaGRP2. PUGNAc treatment increased theO-GlcNAcylation of TaGRP2 and its interaction with VER2 (A). Point mutation in Thr17 significantly reduced the interaction of TaGRP2 with VER2 and the response to pre-incubation with GlcNAc or PUGNAc (B). (C) PUGNAc treatment reduced nuclear-distributed TaGRP2 in vernalized wheat plumules (V28), whereas no change was found in unvernalized (V0). CTD110.6 detectedO-GlcNAcylated TaGRP2. Numbers above indicate relative intensity of TaGRP2 over reference protein (H3 or tubulin) quantified using Image J. (D) Induced expression ofVER2negatively regulates the nuclear accumulation of TaGRP2. The fluorescence ratio between the nuclear and total accumulation in each type of protoplast is shown below the image. Data are mean±s.d. of at least 30 individual cells with three replicates. Scale bar, 10 μm. Figure 4: O -GlcNAcylation of TaGRP2 influences its characteristics. ( A , B ) VER2 predominantly interacts with O -GlcNAcylated TaGRP2. PUGNAc treatment increased the O -GlcNAcylation of TaGRP2 and its interaction with VER2 ( A ). Point mutation in Thr17 significantly reduced the interaction of TaGRP2 with VER2 and the response to pre-incubation with GlcNAc or PUGNAc ( B ). ( C ) PUGNAc treatment reduced nuclear-distributed TaGRP2 in vernalized wheat plumules (V28), whereas no change was found in unvernalized (V0). CTD110.6 detected O -GlcNAcylated TaGRP2. Numbers above indicate relative intensity of TaGRP2 over reference protein (H3 or tubulin) quantified using Image J. ( D ) Induced expression of VER2 negatively regulates the nuclear accumulation of TaGRP2. The fluorescence ratio between the nuclear and total accumulation in each type of protoplast is shown below the image. Data are mean±s.d. of at least 30 individual cells with three replicates. Scale bar, 10 μm. Full size image Following treatment of vernalized wheat plumules with PUGNAc, there was no significant change in the total amount of TaGRP2, whereas the amount of TaGRP2 in the nucleus decreased by about 60% (from 1.00 to 0.42). There was a concomitant increase in TaGRP2 levels in the cytosol (from 1.00 to 1.78; Fig. 4C ). Intriguingly, the PUGNAc-dependent decrease in nuclear TaGRP2 did not occur in unvernalized wheat plumules ( Fig. 4c ). This suggests that O -GlcNAc modification of TaGRP2 influences its sub-cellular localization in a manner involving factors generated during vernalization. 35S::TaGRP2-GFP or 35S::TaGRP2m T17A -GFP together with dexamethasone (DEX) [45] -inducible VER2 were co-transformed into protoplasts generated from wheat plumules after 7 days of cold exposure ( Supplementary Fig. 5a ). In this condition, VER2 is not highly induced ( Supplementary Fig. 5b ), but TaGRP2 had an elevated O -GlcNAcylation level ( Fig. 3d ). Both TaGRP2 and TaGRP2m T17A were localized in the nucleus and in the cytoplasm in the absence of DEX ( Fig. 4D a,d). After inducing expression of VER2 by DEX treatment ( Supplementary Fig. 5b ), nuclear TaGRP2-GFP levels gradually declined: the percentage of nuclear-localized TaGRP2-GFP decreased from about 80 to 30% ( Fig. 4D b,c). No significant change was observed for TaGRP2m T17A -GFP sub-cellular localization during the same time course ( Fig. 4D e,f). Therefore, O -GlcNAc modification of TaGRP2 at Thr17 is important for its interaction with VER2, as well as for vernalization-induced and VER2-dependent nuclear depletion of TaGRP2. TaGRP2 directly binds TaVRN1 and represses its mRNA level RNA in situ hybridization assay revealed TaGRP2 transcript accumulation in the shoot apical meristem (SAM) and young leaves ( Fig. 5a ). This suggests that TaGRP2 overlaps with VER2 and TaVRN1 in those tissues [29] , [46] , raising the possibility that TaGRP2 may participate in regulation of TaVRN1 expression together with VER2. Since TaVRN1 mRNA level increased in TaGRP2 -Ri wheat lines and decreased in TaGRP2 -OE wheat lines ( Fig. 5b ), TaGRP2 may negatively regulate TaVRN1 transcript accumulation. 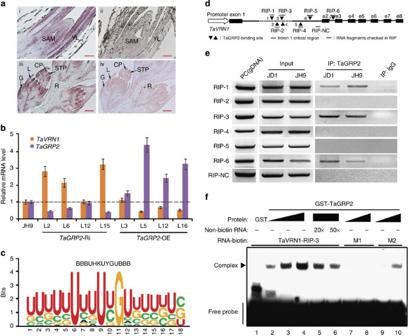Figure 5: TaGRP2 repressesTaVRN1expression by directly binding its pre-mRNA. (a) Expression pattern ofTaGRP2in shoot tips (top) and flower organs (bottom). RNAin situhybridization using aTaGRP2antisense (left) or sense probe (right). SAM, shoot apical meristem; YL, young leaf; G, glume; L, lemma; CP, carpel primordium; STP, stamen primordium; R, rachilla. (b) Transcript accumulation ofTaVRN1andTaGRP2inTaGRP2-OE,TaGRP2-Ri and JH9 plants. The expression levels ofTaVRN1andTaGRP2in wild-type JH9 are set as 1. Relative fold change in the transgenic plants. Data are means±s.d. of three parallel samples. (c) Weblogo of the RNA motif bound by TaGRP2 from RNA library sequences obtained by SELEX. (d) Diagram of the putative TaGRP2-binding sites inTaVRN1. Black triangles indicate the positions of putative TaGRP2-binding sites; dashes show the fragment amplified by RT-PCR after RIP using antibody against TaGRP2. e2–e8, exon 2–exon 8; RIP-NC, RIP negative control fragment. (e,f) Demonstration of direct binding of TaGRP2 toTaVRN1pre-mRNA with conserved binding sites through RIP (e) or RNA-EMSA (f). PC, genomic DNA serves as a positive control. M1 represents RNA probe mutated in the core nucleotide U, U, G; M2 indicates mutation in the adjacent nucleotides. Figure 5: TaGRP2 represses TaVRN1 expression by directly binding its pre-mRNA. ( a ) Expression pattern of TaGRP2 in shoot tips (top) and flower organs (bottom). RNA in situ hybridization using a TaGRP2 antisense (left) or sense probe (right). SAM, shoot apical meristem; YL, young leaf; G, glume; L, lemma; CP, carpel primordium; STP, stamen primordium; R, rachilla. ( b ) Transcript accumulation of TaVRN1 and TaGRP2 in TaGRP2 -OE, TaGRP2 -Ri and JH9 plants. The expression levels of TaVRN1 and TaGRP2 in wild-type JH9 are set as 1. Relative fold change in the transgenic plants. Data are means±s.d. of three parallel samples. ( c ) Weblogo of the RNA motif bound by TaGRP2 from RNA library sequences obtained by SELEX. ( d ) Diagram of the putative TaGRP2-binding sites in TaVRN1 . Black triangles indicate the positions of putative TaGRP2-binding sites; dashes show the fragment amplified by RT-PCR after RIP using antibody against TaGRP2. e2–e8, exon 2–exon 8; RIP-NC, RIP negative control fragment. ( e , f ) Demonstration of direct binding of TaGRP2 to TaVRN1 pre-mRNA with conserved binding sites through RIP ( e ) or RNA-EMSA ( f ). PC, genomic DNA serves as a positive control. M1 represents RNA probe mutated in the core nucleotide U, U, G; M2 indicates mutation in the adjacent nucleotides. Full size image TaGRP2 is predicted to be an RNA-binding protein. To determine the binding motif preference of TaGRP2, we carried out systematic evolution of ligands by exponential enrichment (SELEX) [47] ( Supplementary Fig. 6 ). The RNA motif ‘BBB U HK U Y GU BBB’ was identified as most enriched in the input sequences from the SELEX screen based on MEME2 (ref. 48 ) [48] ( Fig. 5c ; Supplementary Table 4 ). A total of seven such motifs were presented from the 5′ to the 3′-untranslated region in the TaVRN1 gene, all of which were in introns ( Fig. 5d ; Supplementary Table 5 ). RNA immunoprecipitation (RIP) with TaGRP2 antibody followed by real-time PCR (RT-PCR) with specific primers adjacent to the putative binding motifs revealed that TaGRP2 bound to three RNA fragments, RIP-1, RIP-3 and RIP-6 ( Fig. 5e ). Two of them, RIP-1 and RIP-3, are located in the so-called ‘critical region’ of the first intron in TaVRN1 , which is thought to be an important region for regulation of TaVRN1 transcriptional level during vernalization [49] . The third fragment was in the second intron of TaVRN1 . Thus, TaGRP2 binds to the TaVRN1 pre-mRNA in vivo . To test whether TaGRP2 bound to the TaVRN1 RNA fragment in a motif-dependent manner, RNA-electrophoretic mobility shift assay (EMSA) was performed. A 30 nt RNA probe containing the core motif within the RIP-3 (RIP fragment 3) was generated by in vitro transcription and biotin labelled. TaGRP2 bound this RNA probe in a dose-dependent manner ( Fig. 5f ). Mutation of the conserved nucleotides within the core motif of this RNA probe (M1) abolished binding of TaGRP2, while only slightly reduced binding was observed when the adjacent nucleotides were mutated (M2; Fig. 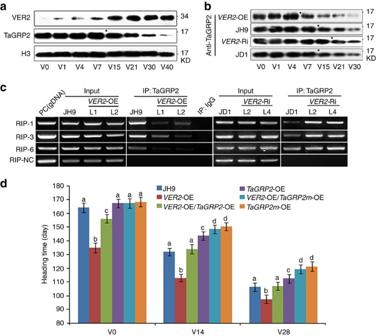Figure 6: VER2 releasesTaVRN1transcriptional repression by TaGRP2 during vernalization. (a) Nuclear protein level of TaGRP2 and VER2 during the course of vernalization in JH9. Star indicates the time point with dramatically reduced TaGRP2 and increased VER2. (b) Nuclear protein level of TaGRP2 during the course of vernalization in JH9, JD1,VER2-Ri (VER2-Ri-L2) andVER2-OE (VER2-OE-L1). Stars show the time point of reduction of TaGRP2. (c) RIP analysis of the amount ofVRN1pre-mRNA bound to TaGRP2 inTaVER2-OE,TaVER2-Ri and JH9 plants. (d) Heading time ofTaVER2-OE, TaGRP2-OE, TaVER2-OE/TaGRP2-OE and wild-type JH9 after different cold exposure times. TaGRP2m stands for point mutation ofO-GlcNAcylation site of TaGRP2 (T17A). Data are means±s.d. of 30 plants for each line. Statistical analyses of multiple comparisons were done by Tukey’s HSD test, different characters indicate statistically significant differences within groups. 5f ; Supplementary Table 6 ). Thus, TaGRP2 directly binds TaVRN1 pre-mRNA in critical region through conserved sequence motif and influences TaVRN1 mRNA accumulation. VER2 releases TaGRP2-mediated repression of TaVRN1 In winter wheat, VER2 protein accumulation is induced after cold exposure and continued to increase later during vernalization. By contrast, the total amount of TaGRP2 did not change dramatically during vernalization ( Supplementary Fig. 7a ). However, the amount of nuclear TaGRP2 began to decrease significantly after 15 days of cold exposure. At the same time, VER2 protein levels dramatically increased in the nucleus ( Fig. 6a ). Furthermore, in VER2 -OE lines, the nuclear accumulation of TaGRP2 started to decrease earlier, after 7 days of cold exposure, whereas it was delayed to 21 days in VER2 -Ri plants ( Fig. 6b ). The total amount of TaGRP2 protein did not show any significant change in either VER2 -OE or VER2 -Ri transgenic plants compared with wild type in response to cold exposure ( Supplementary Fig. 7b ). These data together with the transient expression data ( Fig. 4d ) suggest that VER2 represses nuclear accumulation of TaGRP2 during vernalization in winter wheat. In addition, RIP assays indicated that the relative abundance of the TaVRN1 RNA fragment co-immunoprecipitated with TaGRP2 decreased in VER2 -OE and increased in VER2 -Ri plants regardless of the nuclear protein level of TaGRP2 ( Fig. 6c ). Thus, VER2 also appears to interfere with the binding of TaGRP2 to the target RNA TaVRN1 transcript during the vernalization process. Figure 6: VER2 releases TaVRN1 transcriptional repression by TaGRP2 during vernalization. ( a ) Nuclear protein level of TaGRP2 and VER2 during the course of vernalization in JH9. Star indicates the time point with dramatically reduced TaGRP2 and increased VER2. ( b ) Nuclear protein level of TaGRP2 during the course of vernalization in JH9, JD1, VER2 -Ri ( VER2 -Ri-L2) and VER2 -OE ( VER2 -OE-L1). Stars show the time point of reduction of TaGRP2. ( c ) RIP analysis of the amount of VRN1 pre-mRNA bound to TaGRP2 in TaVER2 -OE, TaVER2 -Ri and JH9 plants. ( d ) Heading time of TaVER2 -OE , TaGRP2 -OE , TaVER2 -OE /TaGRP2 -OE and wild-type JH9 after different cold exposure times. TaGRP2m stands for point mutation of O -GlcNAcylation site of TaGRP2 (T17A). Data are means±s.d. of 30 plants for each line. Statistical analyses of multiple comparisons were done by Tukey’s HSD test, different characters indicate statistically significant differences within groups. Full size image To test whether the repression of TaGRP2 by VER2 functions in flowering regulation in planta , we overexpressed TaGRP2 in the VER2 -OE transgenic plants. VER2 -OE/ TaGRP2 -OE plants flowered significantly earlier than TaGRP2 -OE but later than VER2 -OE ( Fig. 6d ). Thus, repression of TaVRN1 by TaGRP2 was partly released by overexpression of VER2. To test whether this effect depends on the physical interaction between VER2 and TaGRP2, we overexpressed TaGRP2m T17A in wild-type and the VER2 -OE transgenic plants. The flowering time of VER2 -OE/ TaGRP2m T17A -OE plants was similar to that of TaGRP2m T17A -OE plants, indicating that overexpression of VER2 could not overcome the delayed flowering caused by constitutive expression of TaGRP2m T17A ( Fig. 6d ). Thus, regulation of flowering by VER2 is mostly mediated by repressing TaGRP2 activity. The ability of VER2 to repress TaGRP2 is dependent on their physical interaction, which is mediated by O -GlcNAcylation of TaGRP2 at Thr17. As one of the earliest domesticated crops, wheat travelled around the world with human migration. Its broad adaptation is partially due to the available genetic variation in terms of day-length sensitivity and vernalization requirements [8] , [10] . Allelic variation at the TaVRN1 locus is a main determinant of the vernalization requirement [49] , [50] , [51] . One big challenge to understand the molecular basis for vernalization-induced flowering in winter cereals is to elucidate the transcriptional regulation of TaVRN1 . Our report shows that carbohydrate-binding protein VER2, a jacalin lectin, is involved in the induction of TaVRN1 transcription during vernalization. VER2 expression is upregulated after cold exposure in the shoot tips and young leaves [29] , where TaVRN1 functions as a flowering promoter [46] . Overexpression of VER2 could partially substitute for vernalization in acceleration of flowering ( Fig. 1 ), whereas knockdown of VER2 expression led to delayed flowering [29] . TaVRN1 transcript level increased in VER2 -OE and decreased in VER2 -Ri plants. In addition, a change in VER2 levels altered the vernalization requirement for TaVRN1 induction ( Fig. 1 ). VER2 could physically interact with TaGRP2, a negative regulator of flowering in winter wheat ( Fig. 2 ). TaGRP2 transcript presence overlapped with both VER2 and TaVRN1 presence in the shoot apical meristem and in young leaves ( Fig. 5 ). Consistent with this, transcript levels of TaVRN1 increased in TaGRP2 -Ri transgenic plants and decreased in TaGRP2 -OE plants ( Fig. 2 ). Thus, VER2 may interact with TaGRP2 to regulate TaVRN1 transcript abundance and flowering time in winter wheat. In hexaploid wheat, there are 67 VER2-like jacalin-related lectins located in different chromosomes (A, B, D) [52] . Most of them are tissue specific, typically show low expression and are inducible by biotic and abiotic stresses and stress hormones, suggesting that those jacalin-like lectins potentially function in wheat adaptation to various environments (such as long cold winter in the temperate zone). TaGRP2 is a member of the GR-RBP (GRP) family [36] . In Arabidopsis , the orthologue AtGRP7 was proposed to regulate the mRNA processing of genes involved in flowering and stress response through directly binding to their transcripts [53] . Here we showed that TaGRP2 bound to TaVRN1 transcript in a sequence-dependent manner ( Fig. 5 ). The data suggested that TaGRP2 might directly regulate TaVRN1 transcript accumulation. Currently, the mechanism of TaVRN1 induction during vernalization is not clear, however, diverse regulatory events have been identified [8] , [10] , [12] , [54] , [55] , [56] . Before vernalization, the repressive H3K27me3 histone modification is enriched at the TaVRN1 promoter and at the first intron, including the ‘critical region’ in the first intron required for low basal expression level of TaVRN1 (refs 8 , 12 , 34 ). At the onset of vernalization, after a short-term (24 h) cold exposure, TaVRN1 expression increases more than fourfold [54] . Interestingly, this early induction is still observed in TaVRN1 alleles with deletion in the first intron or disruption of a critical vernalization response cis -element called ‘VRN box’ [54] , indicating that it might be mediated by other cis -elements within the promoter region. Consistently, there are multiple Arabidopsis C-repeat binding factor ( AtCBF ) and inducer of CBF1 ( AtICE1 ) putative binding sites in the promoter of TaVRN1 (ref. 56 ). However, this early induction of TaVRN1 is not sufficient to trigger a vernalization response (prolonged TaVRN1 accumulation). To achieve prolonged TaVRN1 accumulation, a histone modification shift from the repressive H3K27me3 to the active H3K4me3 in the promoter and first intron of TaVRN1 may be requried [34] , [55] . Of note, the binding sites of TaGRP2 are within the ‘critical region’ of the TaVRN1 transcript. This suggests the possibility that TaGRP2 repression may need to be overcome for a persistent vernalization response to occur. Consistent with this view, we found that the shift from H3K27me3 to H3K4me3 in the first intron region of TaVRN1 was accelerated in TaGRP2 -Ri plants, accompanied by earlier dramatic accumulation of TaVRN1 ( Supplementary Fig. 8 ). By contrast, the chromatin modification shift and full increase of TaVRN1 mRNA accumulation was delayed in TaGRP2 -OE plants compared with the wild type ( Supplementary Fig. 8 ). Whether TaGRP2 influences histone modifications at the TaVRN1 locus is an interesting question for further research. We have preliminary evidence for the existence of a possible alternatively spliced TaVRN1 transcript or for a possible sense long non-coding RNA that is present in the early stage of vernalization ( Supplementary Fig. 9 ). This transcript initiates from the TaVRN1 transcript start site, contains the entire exon 1 fused to the ‘critical region’ of first intron, including the TaGRP2-binding sites, a region characterized by dynamic histone modification during the vernalization [34] , [35] . In Arabidopsis , the cold-induced long non-coding RNA COLDAIR associates with the PRC2 complex to deposit H3K27me3 at the FLC locus during vernalization [57] . It is possible that the alternatively spliced transcript or long non-coding RNA arising from the TaVRN1 locus may associate with histone modifiers to change the chromatin status of this locus and facilitate its full induction. In Arabidopsis , AtGRP7 binds to its target pre-mRNA to generate an intron-terminating alternatively spliced transcript, which is unstable and degraded through the nonsense-mediated decay pathway [53] , [58] . TaGRP2 might function similarly to regulate the generation or stability of the alternatively spliced TaVRN1 transcript by directly binding to it. Whatever the mechanism, our data suggest that TaGRP2 acts as a repressor that associates with the TaVRN1 transcript prior its full induction by prolonged cold, and before the required changes in histone modifications at this locus in the winter hexaploid wheat. Besides its role in regulation of flowering transition through TaVRN1 , TaGRP2 may also participate in other development process and/or stress response pathways as does its counterpart AtGRP7 in Arabidopsis [59] . Binding motifs for TaGRP2 may be present in additional wheat genes, and future studies aimed at identifying RNA sequences bound by TaGRP2 genome wide could reveal the regulatory potential of this protein. One way by which cells respond to environmental stimuli or change of nutrient status involves dynamic post-translational modification, such as phosphorylation and O -GlcNAcylation, of existing proteins [19] . Our data indicated that the wheat GR-RBP TaGRP2 is subject to O -GlcNAc modification specifically at residue Thr17 during vernalization by presenting different independent pieces of evidence, including immunobloting with CTD110.6 antibody and WGA pull-down, as well as GalNAz labelling ( Fig. 3 ). Due to the limitation of each method, such as cross-reaction with other structure besides O -GlcNAc by CTD110.6 (ref. 41 ), or non-specific linkage (O-link or N-link) for terminal GlcNAc bound by WGA and GalNAz labelling [42] , it is difficult to rule out that TaGRP2 could potentially be modified by other glycan structures. MS analysis is a potential approach to accurately define the linkage and structure in the future. In metazoans, O -GlcNAc modification regulates sub-cellular localization, activity and interactions of proteins [19] , [60] . Many plant proteins are modified by O -GlcNAcylation [25] , [26] , [27] . We found that in wheat, TaGRP2 interacted more strongly with VER2 when its O -GlcNAc modification level was elevated ( Fig. 4 ). This suggests that O -GlcNAc modification of TaGRP2 influences its interaction with VER2, consistent with a requirement for the carbohydrate-binding activity of VER2 for this interaction. In wheat plumules, increased O -GlcNAc modification of TaGRP2 also reduced its nuclear accumulation. This was dependent on prolonged cold exposure, suggesting that other factors induced by vernalization may be needed for the regulation of TaGRP2 sub-cellular localization. In transient expression assays, VER2 accumulation reduced the nuclear localization of wild type, but not the O -GlcNAcylation site T17A-mutated TaGRP2. Thus, O -GlcNAc modification of TaGRP2 may regulate its sub-cellular localization, in a manner dependent on its physical interaction with VER2 during vernalization. Cellular O -GlcNAc levels respond to environmental stresses and modulate the responsiveness of cells to extracellular signalling [60] . Vernalization as a special environmental stress could influence cellular global O -GlcNAc levels [30] . Indeed, glucose treatment can significantly accelerate flowering at an early stage of vernalization, while its effect is reduced at a later stage [61] . Approximately 2–5% of the intracellular glucose enters the hexosamine biosynthetic pathway, which ultimately produces UDP-GlcNAc, the donor for OGT [15] . The concentration of UDP-GlcNAc influences the global cellular O -GlcNAcylation level in animals [60] . During vernalization, cold exposure modulates plant metabolism, which may result in changes to cellular physiological status and content. This in turn may influence the UDP-GlcNAc levels, which are reported to be sensitive to cellular nutrient availability (that is, glucose and/or glucosamine) [62] . A possible consequence could be that O -GlcNAcylation of individual flowering regulators such as TaGRP2 changes during the course of vernalization ( Fig. 3 ). At the same time, as the O -GlcNAcylation of TaGRP2 increased, vernalization-induced effectors such as the lectin VER2 accumulate, which specifically recognize GlcNAc. VER2 interacted with O -GlcNAcylated TaGRP2, reducing its nuclear accumulation and promoting its dissociation from the pre-mRNA of TaVRN1 ( Fig. 6 ). This overcomes the transcriptional repression of TaVRN1 . Consistent with this view, overexpression of VER2 could rescue the delayed flowering caused by overexpression of TaGRP2, but had no effect on overexpression of TaGRP2m T17A , carrying a mutation at the O -GlcNAcylation site ( Fig. 6 ). In this manner, O -GlcNAc signalling contributes to transcript accumulation of TaVRN1 in winter wheat during vernalization, suggesting that a derivative of glucose (that is, UDP-GlcNAc) and/or other may act as signal transduction components at early stages of vernalization to regulate subsequent events during later stages of vernalization. In summary, our work shows that VER2 acts through TaGRP2 to regulate flowering in wheat, and that their interaction is dependent on O -GlcNAcylation of TaGRP2 at Thr17. TaGRP2 directly binds to TaVRN1 pre-mRNA to repress its activation related to histone modification status, and vernalization increases the O -GlcNAc modification of TaGRP2 in the nucleus. VER2, which is induced by long-term cold exposure, recognizes the O -GlcNAc-modified TaGRP2 to repress its accumulation in the nucleus or/and attenuate its binding to TaVRN1 , thereby releasing the repression of TaVRN1 , ultimately promoting flowering ( Fig. 7 ). 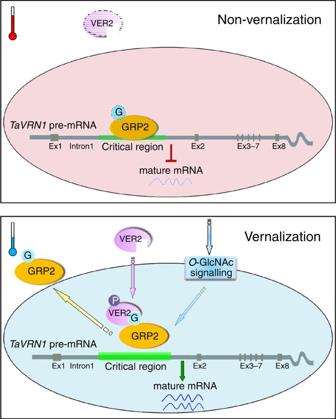Figure 7: Working model for VER2-TaGRP2-mediatedTaVRN1mRNA accumulation during vernalization. Possible model forO-GlcNAc signalling-mediated regulation ofTaVRN1mRNA abundance for flowering transition in winter wheat during vernalization. Under non-vernalization conditions, TaGRP2 bindsTaVRN1and represses its transcript accumulation. Vernalization induces VER2 expression and increases theO-GlcNAcylation level on TaGRP2. Phosphorylated VER2 (VER2-P) translocates into the nucleus and interacts withO-GlcNAcylated TaGRP2 (TaGRP2-G), then releases the repression of TaGRP2 onTaVRN1transcript accumulation. The elliptical ring represents the nucleus, and the area outside represents the cytoplasm. Ex, exon. Figure 7: Working model for VER2-TaGRP2-mediated TaVRN1 mRNA accumulation during vernalization. Possible model for O -GlcNAc signalling-mediated regulation of TaVRN1 mRNA abundance for flowering transition in winter wheat during vernalization. Under non-vernalization conditions, TaGRP2 binds TaVRN1 and represses its transcript accumulation. Vernalization induces VER2 expression and increases the O -GlcNAcylation level on TaGRP2. Phosphorylated VER2 (VER2-P) translocates into the nucleus and interacts with O -GlcNAcylated TaGRP2 (TaGRP2-G), then releases the repression of TaGRP2 on TaVRN1 transcript accumulation. The elliptical ring represents the nucleus, and the area outside represents the cytoplasm. Ex, exon. Full size image Our report presents an example for O -GlcNAc signalling in response to vernalization during the flowering transition in winter wheat. O -GlcNAc signalling may generally be used by plants to coordinate environmental stimulus and endogenous development. Transgenic wheat materials VER2 overexpression ( VER2 -OE), TaGRP2 overexpression ( TaGRP2 -OE) and RNA interference ( TaGRP2 -Ri) transgenic wheat were generated in JH9 accession by microprojectile bombardment-mediated transformation as reported [40] . Briefly, a Chinese winter wheat ( Triticum aestivum ) cultivar JH9 was grown in the field at the Institute of Genetics and Developmental Biology, Chinese Academy of Sciences (IGDB, CAS) experimental station in Beijing, under normal field management conditions. Immature embryos were isolated under aseptic conditions and used in this study. Plasmid pAHC20 that confers the bar gene fused to the ubiquitin promoter and intron 1 from maize. pAHC20 and pUN1301-TaGRP2 or pTCK303-TaGRP2 were used in co-transformation experiments. Plasmid DNA was precipitated onto submicron gold particles (0.6 μm gold, Bio-rad). Particle bombardments were performed using a PDS1000/He particle bombardment system (Bio-Rad, Hercules, CA) with a target distance of 6.0 cm from the stopping plate at helium pressure 1,100 p.s.i. After bombardment, embryos were transferred to callus-induction medium (Murashige and Skoog basal salts including vitamins, 3% sucrose, 2 mg l −1 2,4-dinitrophenylhydrazine (2,4-D), 500 mg l −1 casein hydrolysate and 0.6 g l −1 CuSO4). In the third week after bombardment, all calluses were transferred to selective regeneration medium M1G (Murashige and Skoog basal salts including vitamins, 30 g l −1 sucrose, 0.2 mg l −1 kinetin) containing 5 mg l −1 phosphinothricin (PPT) or 40 mg l −1 hygromycin in the dark. PPT or hygromycin was used in all the subsequent media, including two rounds of regeneration (4 weeks) and two rounds of rooting (half Murashige and Skoog basal salts including vitamins and 3% sucrose, 4 weeks) before being transferred to soil and grown to maturity. Plant materials’ growth condition and vernalization treatment Seeds of winter wheat ( T. aestivum L. cv. JD1, JH9 and VER2 or TaGRP2 transgenic lines) were surface sterilized in 2% NaClO for 20 min, then rinsed overnight with flowing water. After that, the seeds were germinated on moist filter paper under gradient time (1, 4, 7, 15, 21, 30 and 40 days, as V1, V4, V7, V15, V21, V30, V40) of 4 °C treatment in the dark (V), or grown at 25 °C for 3 days (V0). Then, transferred to soil and grown in greenhouse (20–22 °C, 16 h light/8 h dark). For the condition of natural vernalization, seeds without cold exposure were sowed in the field of Botanic Garden, Institute of Botany, CAS, Beijing, China, at the beginning of October every year. They experienced the natural vernalization during winter, and flowered in the next spring. Protein isolation by chromatography Total proteins were extracted from wheat plumules of 2 g after 20 days of cold (4 °C) exposure in the dark. After quantification by Bradford assay, about 20 mg proteins was isolated by ion-exchange chromatography (DEAE-cellulose). Fractions were collected and isolated by SDS–PAGE, followed by immunoblotting with VER2 antibody. Samples containing VER2 were concentrated, pooled and further isolated using size-exclusion chromatography (Super DEX 200). Fractions were collected, isolated by SDS–PAGE and immunoblotted with VER2 antibody. Specific bands co-segregating with VER2 were in-gel digested with trypsin and further identified using a MS (LTQ). The isolated peptides were searched in the database from NCBI (green plants). Protein interaction analysis Co-IP and BiFC assays were performed in protoplasts generated from wheat plumules. Briefly, FLAG-VER2 was co-expressed with TaGRP2-GFP or GFP, and after transformation, protoplasts were collected and ground in nuclear extract buffer, filtered and centrifuged. The supernatant was incubated with anti-GFP antibody coupled to protein A/G sepharose beads, the beads were washed four times with wash buffer and bound proteins were eluted with buffer containing 1% SDS for immunoblotting with FLAG antibody. For BiFC assays, constructs for expression of VER2-YFP (yellow fluorescent protein) NE , TaGRP2-YFP CE , VER2-YFP CE and TaGRP2-YFP NE were generated and transformed into protoplasts. Yellow fluorescent protein (YFP) fluorescence was visualized using a confocal scanning microscope 40–48 h after infiltration. RNA in situ hybridization Wheat plumules of seedlings and young panicles were fixed in a solution of 50% (v/v) ethanol containing 3.7% (v/v) formaldehyde and 5% (v/v) acetic acid at room temperature for 16 h. The fixed tissues were dehydrated in a graded ethanol series, cleared with xylene and embedded in Paraplast (Sigma). Sections (10 μm) were placed on poly-lysine-coated slides (Sigma). After dewaxing and rehydrating, the sections were digested for 30 min at 37 °C in a solution containing 100 mM Tris–HCl (pH 7.5), 50 mM EDTA and 5 μg ml −1 proteinase K; acetylated by incubating in 0.25% acetic anhydride in 100 mM triethanolamine–HCl (pH 8.0), for 5 min; dehydrated in a graded ethanol series to 100% and dried at room temperature. Hybridization in situ was carried out according to previous publication [63] . Briefly, the antisense and sense RNAs of TaGRP2 were labelled with digoxigenin (DIG) through in vitro transcription of linearized pTaGRP2 (DIG Northern Starter Kit; Roche, Mannheim, Germany) and hydrolyzed to a mean length of ~100 bases in carbonate buffer at 60 °C. Hybridization was carried out at 42 °C overnight with a solution containing 0.2 ng μl −1 probe, 50% formamide, 300 mM NaCl, 10 mM Tris–HCl (pH 7.5), 1 mM EDTA, 5% dextran sulphate, 1% blocking reagent (Roche), 150 μg ml −1 transfer RNA and 500 μg ml −1 poly(A). Labelled probe was detected through alkaline phosphatase coupled to anti-DIG antibody Fab fragments and 4-nitroblue tetrazolium chloride/5-bromo-4-chloro-3-indolyl-phosphate (Roche). When the colour reaction was complete, the section was dehydrated in an ethanol series, cleared in xylene and mounted in Canada gum. Sections were observed and photographed by bright-field microscopy. 1D/2D SDS–PAGE and immunoblot analysis Total protein or nucleus and cytoplasm fractions were extracted and quantified by Bradford assay, proteins of 20 μg per lane were separated on 12% (for tubulin and CTD110.6 antibodies) or 16% (for TaGRP2 and histones) SDS–PAGE gels and electroblotted onto polyvinylidene difluoride membranes. Immunoblotting was done by using the enhanced chemiluminescence (ECL) system [30] . For 2D electrophoresis, dry strip gels (7 cm, pH 4–7, Amersham) were used. Uncropped immunoblot images are shown in Supplementary Fig. 10 and 11 . Sub-cellular proteins’ fractionation Nuclear and cytoplasmic protein fractions were isolated as described [64] . Briefly, plant material was ground in extraction buffer and filtered through Miracloth (Calbiochem) to obtain the total extract, and then centrifuged at 3,000 g . The supernatant (cytoplasmic fraction) was removed and stored on ice until use. The pellets were further washed with a re-suspension buffer and then reconstituted as the nuclear fraction. Immune detection of H3 (Histone 3) and tubulin was used to confirm the fractionation of nucleus and cytoplasm, respectively. WGA affinity protein purification Lectin affinity chromatography was carried out with WGA-agarose beads (Amersham Biosciences) using 2.0–4.0 mg total protein extract. Lectin beads were incubated with protein extracts for 1 h at room temperature. Glycosylated proteins were eluted from the beads with 1 M GlcNAc for 10 min at room temperature. Immunoprecipitates were subjected to SDS–PAGE (15%), and immunoblot analyses were performed using TaGRP2 antibody or O -GlcNAc antiserum. RNA-EMSA RNA probes were generated in vitro using a T7 high-yield transcription kit (Invitrogen). Biotin was added to the 3′ end of RNA probes using the RNA 3′ End Biotinylation Kit (Pierce). RNA-EMSA was performed according to the kit instructions (Pierce). Purified RNase-free GST-TaGRP2 was used. All probe sequences, including those for mutations, are listed in Supplementary Table 6 . RIP and RT-PCR RIP was performed as previously indicated [65] , [66] , with a little modification. Briefly, 3 g wheat seedling was harvested and cross-linked by 0.5% formaldehyde. Plant material was ground and suspended in 15 ml Honda buffer supplemented with 8 U ml −1 RNase inhibitor, filtered through two layers of Miracloth (Calbiochem) and centrifuged at 3,000 g for 7.5 min at 4 °C. The pellet was re-suspended in 500 μl nuclei lysis buffer+160 U ml −1 RNase inhibitor. Sonicate and centrifuge the samples, transfer the supernatant to the fresh tubes. Measure DNA concentration in the samples and ensure that nucleus protein concentrations are similar in all samples. Prepare 100 μl aliquots of the samples. Dilute the samples tenfold with chromatin immunoprecipitation (ChIP) dilution buffer+350 U ml −1 RNase inhibitor. Immunoprecipitation was done by adding 2 μl TaGRP2 antibody (purified mouse polyclonal antibody) and 20 μl Protein A agarose/Salmon Sperm DNA (Upstate, 16–157) pre-washed three times by binding/washing buffer to the solution. Pre-immune mouse serum was used as negative antibody control. After incubating on a rotator for 3 h at 4 °C, wash beads four times with 1 ml binding/washing buffer+40 U ml −1 RNase inhibitor and elute the protein–RNA complex with 50 μl RIP elution buffer+40 U ml −1 RNase inhibitor. Then, the protein was degraded by proteinase K, and RNA was extracted by acidic phenol/chloroform and precipitated by ethanol supplemented with 3 M NaAc, pH 5.2, and 5 mg ml −1 glycogen (Ambion). Wash the pellet with 70% ethanol, air-dry and dissolve in RNase-free water. RNA sample was incubated with DNase I to digest the DNA containment. For identification and quantification by RT-PCR, RNA samples were polyadenylated at 37 °C for 30 min with 5 U poly(A) polymerase (Takara). Poly(A)-tailed RNA was recovered by phenol/chloroform extraction and ethanol precipitation. A 5′ adapter (GeneRacer RACE ready cDNA kit, Invitrogen) was ligated to poly(A)-tailed RNA using T4 RNA ligase (Invitrogen) and the ligation products were recovered by phenol/chloroform extraction followed by ethanol precipitation. Reverse transcription was performed using GeneRacer Oligo d(T) primer (SSIII) with 200 U of SuperScript III reverse-transcriptase (Invitrogen). The first-round PCR was carried out for 22 cycles with GeneRacer 5′/3′ primers. The PCR products were separated on 1% agarose gel, and DNA smear from 200 to 800 bp was recovered and diluted 20-fold to be used as template for the secondary-round PCR with GeneRacer-nested 5′/3′ primers. The PCR products were separated on 1% agarose gel, and DNA smear from 150 to 800 bp was recovered and diluted 50-fold to be used as template for detection of interested gene fragments with gene-specific primers ( Supplementary Table 6 ). For qualification and quantification, the genome DNA served as positive control for PCR and input samples (without immunoprecipitation) were used for equal loading. ChIP assay ChIP experiments were performed using winter wheat seedlings (JH9) treated by gradient time of cold exposure [67] . Antibodies with specificity to H3K4me3 or H3K27me3 were used to immunoprecipitate the chromatin. The amount of immunoprecipitated TaVRN1 chromatin was determined by RT-PCR on different regions of TaVRN1 locus as shown in Fig. 1d . Primer sequences are listed in Supplementary Table 6 . The relative abundance was normalized to the amount of DNA immunoprecipitated by antibody specific to H3. Protoplast transformation Plasmids of 35S::TaGRP2-GFP , 35S::TaGRP2m-GFP , 35S::VP16-GR and 8OP::VER2 were purified by the use of Tiangen or Qiagen kits according to the manufacturer’s protocols. The wheat protoplast transformation by polyethylene glycol (PEG) was according to the previous reports [45] , [68] , with some modification. Wheat seeds were first sterilized, grown on 1/2 MS medium under light for 3 days and then transferred to the dark for 7–10 days. Sheath and stem tissues were cut into 0.5 mm pieces with the use of sharp razors. Tissues were immediately incubated in enzyme solution (0.6 M mannitol, 10 mM MES, pH 5.7, 1.5% cellulase RS, 0.75% macerozyme R10, 0.1% bovine serum albumin, 1 mM CaCl 2 and 5 mM β-mercaptoethanol) for 4 h in the dark with gentle shaking (40 r.p.m.). After incubation, one volume of W5 solution (154 mM NaCl, 125 mM CaCl 2 , 5 mM KCl, 2 mM MES, pH 5.7) was added. Protoplasts were passed through a 35-μm nylon mesh filter. The solution was centrifuged for 5 min at 300 g to pellet the protoplasts, and then washed again with W5. Cells at 2 × 10 6 cells ml −1 were re-suspended in Mmg solution (0.4 M mannitol, 15 mM MgCl 2 , 4 mM MES, pH 5.7) for PEG-mediated transformation and kept on ice for 30 min. For transformation, 40% PEG (0.2 M mannitol, 100 mM CaCl 2 , 40% v/v PEG4000, Fluka) was added to the protoplasts for 15 min. Cells were washed 1 × with 10 volumes of W5 and then re-suspended in W5. All of the experiments were performed at room temperature. Cells were then incubated at 28 °C in the dark overnight. For DEX treatment, 10 μM DEX was added to the protoplasts 8 h after transfection and incubated for 2–4 h. Observation and quantification of fluorescent protein signal GFP/YFP fluorescence was visualized using a confocal microscope (Leica TCS SP5, German) with an argon laser (488 nm); the auto-fluorescence of chloroplasts also appeared at this excitation wavelength. Images of fluorescence at different layers along the z axis were collected and overlaid to give a full view of the GFP/YFP signal. Bright field images were captured at the proper layers of the z axis to show the position of the whole protoplast cells, respectively. Quantification of the fluorescent protein signal was performed using Image J ( http://rsb.info.nih.gov/ij ). To calculate the ratio of the nucleus to total signals of TaGRP2-GFP for each cell, nucleus positional area and GFP signal intensity were measured and divided by the total GFP signal of the whole cell. A representative image of each transformant is shown in Fig. 4d . The numbers indicate the relative nuclear-distributed ratio of TaGRP2-GFP. This experiment was carried out for three biological replicates, with each sample consisting of at least 30 cells analysed, and the signal intensity is presented as mean±s.d. Site-directed mutagenesis Mutation of TaGRP2 (Thr17 Ala) was generated by using the QuikChange Site-Directed Mutagenesis Kit (#200519, Stratagene) according to the manufacturer’s protocols. The mutated product was confirmed by sequencing with three individual clones. Primers used are listed in the Supplementary Table 6 . Primers and antibodies Primers used in this study were purchased from Invitrogen Company ( Supplementary Table 6 ). All the antibodies used in this study are described in Supplementary Table 7 . How to cite this article: Xiao, J. et al . O -GlcNAc-mediated interaction between VER2 and TaGRP2 elicits TaVRN1 mRNA accumulation during vernalization in winter wheat. Nat. Commun. 5:4572 doi: 10.1038/ncomms5572 (2014).